Twinning-like lattice reorientation without a crystallographic twinning plane Twinning on the plane is a common mode of plastic deformation for hexagonal-close-packed metals. Here we report, by monitoring the deformation of submicron-sized single-crystal magnesium compressed normal to its prismatic plane with transmission electron microscopy, the reorientation of the parent lattice to a ‘twin’ lattice, producing an orientational relationship akin to that of the conventional twinning, but without a crystallographic mirror plane, and giving plastic strain that is not simple shear. Aberration-corrected transmission electron microscopy observations reveal that the boundary between the parent lattice and the ‘twin’ lattice is composed predominantly of semicoherent basal/prismatic interfaces instead of the twinning plane. The migration of this boundary is dominated by the movement of these interfaces undergoing basal/prismatic transformation via local rearrangements of atoms. This newly discovered deformation mode by boundary motion mimics conventional deformation twinning but is distinct from the latter and, as such, broadens the known mechanisms of plasticity. Deformation twinning (DT) is a major mode of plastic deformation for metals with the hexagonal-close-packed (HCP) structure [1] , [2] , [3] , [4] , [5] , [6] , owing to their very limited number of slip systems available for dislocation glide. However, twinning mechanisms for such HCP metals are much less understood when compared with face-centred-cubic metals, for which twin boundary (TB) migration is well established to be accomplished via the glide of Shockley partial dislocations on the twinning plane [1] , [5] , [7] . For the DT that is prevalent in almost all HCP metals, both mobile disconnections [8] , [9] , [10] , [11] , [12] , [13] , [14] , [15] acting as twinning dislocations and atomic shuffling [16] , [17] , [18] , [19] , [20] , [21] have been argued to be the dominating and rate-limiting element. These debates suggest that there is a pressing need to better understand the details of the deformation dynamics in HCP-structured metals experimentally. In this work, we choose to study submicron-sized single-crystal pure magnesium. On one hand, submicron-sized samples are sufficiently thin to be electron transparent, which allows us to monitor and record the nucleation and propagation of DT at high spatial resolution. On the other hand, submicron-sized crystals may be much stronger than their bulk counterparts, according to the well-established tenet of ‘smaller is stronger’. Consequently, our study may reveal unusual deformation mechanisms under high-stress conditions, which may also exist in bulk magnesium due to local stress concentrators such as grain boundary or precipitates. The samples were fabricated using focused ion beam (FIB) micromachining and then tested inside a transmission electron microscopy (TEM) employing the Hysitron PI95 Picoindenter [22] , which enables one-to-one correspondence between the external applied stress/strain and the microstructure evolution of the deforming material. The sample/loading orientation is shown schematically in Fig. 1a . When viewed along the direction, the angle between the trace of the plane and the loading axis is 43.1°. The DT is expected to be activated in this configuration when the specimen is compressed. 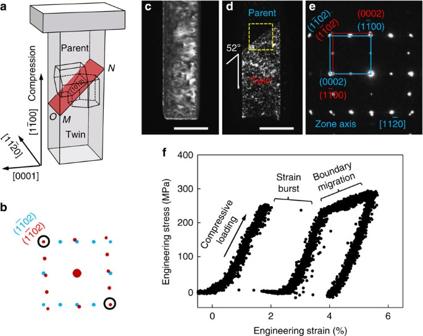Figure 1:In situcompression test on a submicron-sized single-crystal Mg pillar. (a) Schematic illustration of the crystal, compression-loaded inorientation. Theplane is highlighted in red. (b) SADP for idealtwins. (c,d) Dark-field TEM images showing the pillar before and after loading, respectively. Scale bars, 400 nm. (e) SADP taken from the framed area, demonstrating thatdiffraction spots are separated instead of overlapping with each other. The zone axis isfor parent lattice. (f) The corresponding stress–strain curve. Figure 1: In situ compression test on a submicron-sized single-crystal Mg pillar. ( a ) Schematic illustration of the crystal, compression-loaded in orientation. The plane is highlighted in red. ( b ) SADP for ideal twins. ( c , d ) Dark-field TEM images showing the pillar before and after loading, respectively. Scale bars, 400 nm. ( e ) SADP taken from the framed area, demonstrating that diffraction spots are separated instead of overlapping with each other. The zone axis is for parent lattice. ( f ) The corresponding stress–strain curve. Full size image ‘Deformation twinning’ For the testing condition in Fig. 1a , ‘deformation twinning’ appeared to be all that had happened, at the first glance. One typical example is shown in Fig. 1c–f . The initial dimensions of this sample are 400 × 500 × 1,600 nm 3 ( Fig. 1c ). During compression, a strain burst (~2%) set in at ~250 MPa ( Fig. 1f ), which is much higher than the yield strength of bulk single-crystal magnesium with same orientation. At the same time, a twin-like feature formed. The fast release of the accumulated elastic energy made it difficult to differentiate the ‘twin’ nucleation and the following quick growth process. However, the measured strain generated by the ‘twinned’ volume during the strain burst agrees well with that predicated by theoretical calculations. As the test was controlled under a fixed displacement rate, the flat punch probe detached from the sample at the moment of the burst, which in turn slowed down and stopped the ‘twin’ growth temporally. Correspondingly, an apparently straight boundary running across the gauge part of the sample can be seen clearly. After the flat punch probe caught up with the sample to continue the compression, this boundary migrated continuously until the end of the programmed total displacement ( Supplementary Movie 1 ). The trace of the boundary looks quite smooth and straight ( Fig. 1d ) at this magnification, as expected for the TB of the DT. The DT is supposed to generate a plastic strain of ~6%; here the strain burst and the following boundary migration swept about 60% of the sample in its length direction ( Fig. 1d ), such that the plastic strain generated should be ~3.6%, as found in the experiment data in Fig. 1f . However, a close examination revealed that several features are inconsistent with deformation twining. First, the inclination angle (52°) of the boundary shows a pronounced deviation from that expected from the plane, by as much as 9°. Second, for DT, the diffraction spots should overlap in the corresponding selected area diffraction pattern (SADP), as shown in Fig. 1b . However, the SADP acquired across the boundary shows that the diffraction spots are actually separated ( Fig. 1e ), and the angle between the basal planes of the parent and the deformed regions is close to 90° rather than the 86.3° expected for DT. It thus appears that while we seem to have activated DT, the reoriented lattice in the deformed region does not hold a rigorously crystallographic (rational) orientational relationship with the parent lattice as expected for twinning. 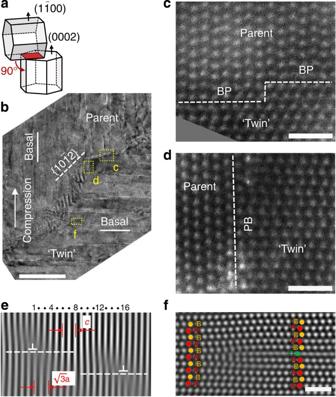Figure 2: Atomic structure of the deformation boundary. (a) Schematic showing the orientation relationship between the ‘twin’ and its parent lattice. (b) High-resolution TEM image showing the rugged boundary (see atomic resolution images incandd), with stacking faults on both sides of the boundary. Scale bar, 50 nm. (c,d) Scanning TEM images of typical basal/prismatic interface and prismatic/basal interface, respectively. (e) One-dimensional lattice fringe image obtained by applying a fast Fourier transform filtering process showing two misfit dislocations at the basal/prismatic interface. (f) A noise-filtered image of a stacking fault in the deformed volume. Scale bars, 1 nm (c,d,f). The e-beam direction is. Basal/prismatic interfaces Figure 2a schematically illustrates the actual orientational relationship as indicated by the SADP in Fig. 1e . To characterize the atomic structure of the boundary (marked by red colour), the sample shown in Fig. 1d was further thinned and examined inside a spherical aberration-corrected TEM. The high-resolution TEM observations reveal that the straight boundary in Fig. 1d in fact has a rugged structure ( Fig. 2b ) throughout the entire boundary. The Moiré fringes observed at the boundary areas are a result of the overlap between two crystals, the parent and the ‘twin’ regions. On the atomic level, the ‘twin’/parent boundary actually consists of two types of interfaces: basal/prismatic interface ( Fig. 2c ) and prismatic/basal interface ( Fig. 2d ). The existence of such interfaces was predicted recently by computer simulations [23] , [24] . These two types of interfaces, perpendicular to each other, constitute a stepped boundary between the deformed and undeformed regions. In other words, while TBs are present in some local regions, along the boundary the segments are few and far between. Zooming in down to the atomic level, the majority of the boundary is instead composed of (pairs of) basal/prismatic and prismatic/basal interfaces. This is also true for samples deformed in tensile tests (loaded along the [0001] direction), see Supplementary Fig. 1 . There is no rational crystallographic orientational mirror symmetry established across these basal/prismatic interfaces. The boundary is therefore not a TB per se , and the 90° twin-like orientation relationship described in the preceding paragraph is established via reorientation actions at the basal/prismatic interfaces rather than on a crystallographic, invariant twinning plane. However, considering that the atomistically wavy boundary appears ‘straight’ at low magnifications ( Fig. 1 ) and the orientation relationship between the parent and ‘twin’ regions is close to that in DT, we refer the two regions in all the figures of this paper as the parent lattice and the ‘twin’ lattice, respectively. Figure 2: Atomic structure of the deformation boundary. ( a ) Schematic showing the orientation relationship between the ‘twin’ and its parent lattice. ( b ) High-resolution TEM image showing the rugged boundary (see atomic resolution images in c and d ), with stacking faults on both sides of the boundary. Scale bar, 50 nm. ( c , d ) Scanning TEM images of typical basal/prismatic interface and prismatic/basal interface, respectively. ( e ) One-dimensional lattice fringe image obtained by applying a fast Fourier transform filtering process showing two misfit dislocations at the basal/prismatic interface. ( f ) A noise-filtered image of a stacking fault in the deformed volume. Scale bars, 1 nm ( c , d , f ). The e-beam direction is . Full size image The basal/prismatic and prismatic/basal interfaces are semicoherent because of the lattice mismatch, as confirmed by the existence of misfit dislocations at the interfaces: the dislocation separation spacing is counted to be 15 lattice fringes ( Fig. 2e ). In many regions, the basal plane of the parent lattice is not exactly parallel to the prismatic plane of the ‘twin’ lattice: this is a result of local strains near the boundary or other defects (see Supplementary Note 1 and Supplementary Table 1 ). Basal stacking faults were observed on both sides of the boundary, but the density is much lower in the parent region than that in the ‘twinned’ region. Figure 2f shows a high-resolution image of one of such stacking faults. ‘Twin’ propagation We found that the lattice reorientation is reversible when the loading direction was switched from tensile to compression. Most surprisingly, we found that the ‘twin’ boundary can propagate without an obvious twinning shear, as shown in Fig. 3 . This sample was initially in dog-bone shape and was deformed under uniaxial tension along the [0001] direction. This led to the parent-to-‘twin’ conversion, much like the case of compression in the direction perpendicular to [0001] (the scenario described in Fig. 1 ). We then took the ‘twinned’ sample out of the TEM and made it into a pillar with FIB by chopping off the T-shaped free end ( Fig. 3a ). The pillar was then subjected to programmed compressive loading ( Fig. 3b ), now along the direction perpendicular to the (newly formed) prismatic plane. The orientation is now the same as that in Fig. 1 and the only difference is that the sample has already gone through the basal/prismatic transformation once to reach this orientation. The ensuing deformation is therefore a reverse transformation, or ‘de-twinning’, process (see diffraction patterns in Supplementary Fig. 2 ). As expected, following the nucleation of ‘de-twinning’ at the free end, the deformation boundary propagated gradually towards the root part of the pillar along with compression deformation, with the moving boundary nearly perpendicular to the loading axis. Most interestingly, the ‘de-twinned’ part ( Fig. 3e ) uniformly swelled towards both sides of the pillar, rather than sheared in a specific direction, during the entire deformation process ( Supplementary Movie 2 ). The observation in Fig. 3 and Supplementary Movie 2 demonstrates that the propagation of the boundary is not coupled to simple shear, but rather, tetragonal compression. This is in sharp contrast with any DT mechanism where the lattice reorientation is carried predominantly by twin shear. 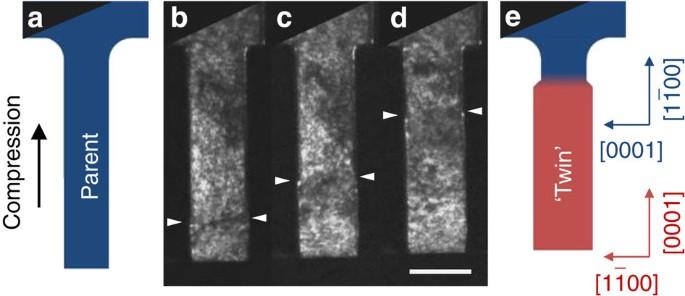Figure 3: Basal/prismatic interfaces mediated boundary migration. PanelsaandeSchematically showing the sample condition before and after the compression test, respectively. Panelsb–dare snapshots extracted from the recorded movie showing the boundary (marked by a pair of white arrows) movement with time. Note that the sample swells towards both sides and shrink in the loading direction. Scale bar, 400 nm. Figure 3: Basal/prismatic interfaces mediated boundary migration. Panels a and e Schematically showing the sample condition before and after the compression test, respectively. Panels b – d are snapshots extracted from the recorded movie showing the boundary (marked by a pair of white arrows) movement with time. Note that the sample swells towards both sides and shrink in the loading direction. Scale bar, 400 nm. Full size image Twinning-like lattice reorientation To recap, the interesting finding from our experiments is that in many regions a transformation process can take over to directly convert basal plane to prismatic plane, and vice versa . Although the chain of transformation events at numerous basal/prismatic and prismatic/basal interfaces achieves a crystal reorientation that appears not far off from the DT, a close look probing the boundary reveals that this net result is accomplished through a distinctly different mechanism. While DT requires a single, crystallographic mirror plane (the invariant plane), the new deformation mode relies on coordinated motion of basal/prismatic interface couples, without establishing crystallographic mirror orientational relationship right across the interfaces. The combination of a large number of basal/prismatic interfaces intermixed with prismatic/basal interfaces, with varying segment lengths, can lead to different inclination angles when viewed from a distance, including those (such as 52°) that deviate considerably from what is known for the DT. Our newly discovered deformation mode mimics conventional DT but is distinct in two important aspects. A textbook definition of DT is that it achieves simple shear of a crystal, while possessing a crystallographic invariant plane or twinning plane. Our deformation mode can achieve tetragonal compression ( Supplementary Movie 2 ) instead of simple shear, and it does not possess a crystallographic characteristic plane seen at the larger-length scale. In term of the atomistic mechanism for lattice reorientation, neither the well-known pole mechanism [1] , [3] nor the disconnection mechanism [8] , [9] , [10] , [11] , [12] , [13] , [14] , [15] for DT can explain the nucleation, propagation and structure of the deformation boundary observed in this work. While further studies are clearly needed, in the following we discuss the mechanism in a qualitative manner. Two HCP frames are schematically shown in Fig. 4a , with one HCP embryo parasitizing inside another. The red and blue symbols outline the ‘twin’ and its parent lattice, respectively. The two structures are rotated 90° relative to one another. When a sufficiently high compressive stress is applied normal to the prismatic plane, the blue HCP can transform to the red one. The arrows indicate the possible route for the required atomic rearrangements. The prismatic planes in the parent body transform into the basal planes of the new lattice, creating the basal/prismatic interface with misfit dislocations. Such a mechanism and the migration of the basal/prismatic interfaces can in fact be visualized in molecular dynamics (MD) simulations ( Fig. 4b–e ). When a 1.5-GPa compressive stress is applied perpendicular to a basal/prismatic interface, we observe a disconnection with a height of two atomic layers ( Fig. 4c ) moving upwards with the step of 2 n atomic layers (where n is an integer). Concurrent with this DT, the nearby basal/prismatic interface also migrates, with accompanying formation of prismatic/basal interface, which is what is observed in our experimental samples. 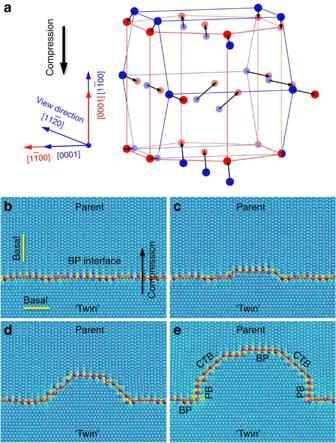Figure 4: Atomic view of the basal/prismatic transformation. (a) The parent HCP frame (blue) and ‘twin’ HCP frame (red) as well as their possible transformation route via shuffling atomic rearrangements. The right-bottom atoms (half blue and half red) were chosen to be the reference point. (b–e) MD simulations showing the migration of basal/prismatic (BP) and prismatic/basal (PB) interfaces under compressive loading. The coherent TB (CTB) is present despite of the 90° (rather than 86°) lattice orientational relationship, because there are coexisting dislocations at the boundary. SeeSupplementary Informationfor simulation details. Figure 4: Atomic view of the basal/prismatic transformation. ( a ) The parent HCP frame (blue) and ‘twin’ HCP frame (red) as well as their possible transformation route via shuffling atomic rearrangements. The right-bottom atoms (half blue and half red) were chosen to be the reference point. ( b – e ) MD simulations showing the migration of basal/prismatic (BP) and prismatic/basal (PB) interfaces under compressive loading. The coherent TB (CTB) is present despite of the 90° (rather than 86°) lattice orientational relationship, because there are coexisting dislocations at the boundary. See Supplementary Information for simulation details. Full size image The next question to address is why the basal/prismatic transformation mode becomes prevalent in our submicron samples. We note that, as expected from the well-established tenet of ‘smaller is stronger’, the stress required for activating twinning dislocations on planes will increase with decreasing sample size [25] . The availability of disconnections assisting DT is limited in small-volume samples. Since our crystal is compressed perpendicular to its prismatic plane, the high normal stress facilitates the short-range rearrangement of atoms to form a new basal plane. This may render basal/prismatic conversion kinetically more favourable than the motion of the coherent interface, although the latter has a lower interfacial energy (125 mJ m −2 ) relative to the basal/prismatic interface (170 mJ m −2 ). As such, the basal/prismatic conversion at numerous basal/prismatic interfaces assists and accommodates the DT to produce plastic strain. Our submicron-sized sample provides a high free-surface-to-volume ratio, possibly making it easier to accommodate the strains associated with the lattice reorientation and the misfit dislocations generated at the basal/prismatic interface. However, it is noteworthy that the basal/prismatic interfaces were also observed in a bulk magnesium alloy deformed under high strain rates (see Supplementary Discussion and Supplementary Fig. 3 ). This suggests that the basal/prismatic conversion mode may be activated under many high-stress conditions and thus be of general importance in HCP metals. The newly revealed transformations at the basal/prismatic interfaces may also have implications for alloy design. For example, basal/prismatic interfaces may have different propensity for trapping solute atoms [26] when compared with coherent twin boundaries. The propagation of basal/prismatic interface may be less sensitive to precipitates that are traditionally important for age hardening [27] . Before closing, we point out several open questions for future exploration. First, Yu et al. [28] carried out similar tests on single-crystal magnesium in a similar size range, but they observed populous coherent twin boundaries. Further experiments are necessary to clarify whether the difference is related to compositional difference. Second, copious stacking faults parallel to the basal planes have been observed on both sides of the boundary (in the deformed and undeformed regions). It remains to be seen whether these stacking faults can improve strain hardening [29] , thereby improving the ductility of magnesium alloys. Finally, the transformation at the moving basal/prismatic interfaces can be regarded as a special case of stress-driven grain boundary migration [30] , [31] , [32] but disagreeing with the conventional theory of shear-coupled grain boundary motion. Our new mechanism at the sweeping boundary ( Supplementary Movie 2 ) produces a sizable plastic strain of tetragonal compression character instead of simple shear. TEM and in situ mechanical testing The submicron-sized samples were fabricated via FIB micromachining. In situ mechanical test was conducted using a Hysitron PicoIndenter (PI95) inside a JEOL 2100FEG TEM (200 keV). More than 30 tests were conducted successfully on 27 samples (for more details see Supplementary Table 2 and Supplementary Note 2 ). The strain rate was of the order of 10 −3 s −1 . To investigate the atomic structure of the boundaries, the deformed sample was further thinned by using M1040 Nano Mill (Fischione Inc). The atomic resolution TEM images were acquired using an ARM200F spherical aberration-corrected TEM, under scanning TEM (200 keV) imaging mode. Measures taken to minimize the potential artefacts We have designed our experiments carefully to minimize the effects from the following factors: sample taper, stress concentrations, misalignment and FIB effects. In the following, we will detail the measures we have adopted. (1) Taper: to minimize the taper, we used FIB to fabricate the pillar with square cross-section and carefully adjusted the cutting angles in the final steps. As shown in Supplementary Fig. 4 , the taper angle for as-fabricated samples is quite small. (2) Stress concentration: stress concentration did exist at the contact interface between the probe and pillar, which was evidenced by the fact that the apparent nucleation stress observed in pillar samples is much lower than that in ‘dog-bone’ samples ( Supplementary Fig. 5 ). This is conceivable because it will be very difficult to make the free-end surface of the tested sample exactly parallel to probe surface. Comparably speaking, the ‘dog-bone’ shape samples do not have such drawbacks. Therefore, we employed both pillar and ‘dog-bone’ samples to confirm that our findings are the intrinsic properties of the tested material instead of artefacts resulted from the stress concentration. The fact that boundary migration stresses in both ‘dog-bone’ samples and pillars are on the same level suggests that stress concentration resulted from the contact interface has much less effect on boundary migration. (3) Misalignment: all our in situ tests have been designed carefully under the guidance of electron beam. Therefore, misalignment is unlikely to play a significant role. (4) The following measures were adopted to minimize the effect from FIB. First, we fabricated the sample via glancing cutting on the lateral surface. Second, a low-energy (5 keV) ion beam was used to clean the sample surface and minimize the damage layer thickness. TEM observation confirmed that the FIB influenced layer was usually less than a few nanometres. As our samples have dimensions of about 400 nm, the effects from FIB should be insignificant. MD simulation Atomistic simulations were performed for Mg with empirical interatomic potentials [33] . A bicrystal model is constructed with periodic boundary conditions in all three dimensions. Two identical semicoherent basal/prismatic interfaces are created in the x–z plane. The equilibrium, relaxed model has the dimensions of 49.8 nm in the x direction, 15.98 nm in the z direction and 15 nm for each crystal in the y direction. Owing to the mismatch of lattices in the x direction ( κ is the c/a ratio), the semicoherent basal/prismatics contain an array of misfit dislocations, which can be described as with respect to the prismatic plane or with respect to the basal plane. The average spacing is 8.3 nm, suggesting that the misfit dislocation would not be present in short basal/prismatic interfaces. We performed MD at a temperature of 10 K under a compressive stress perpendicular to the basal/prismatic interface plane. During compression, the nucleation and motion of interface disconnections commence at a compressive stress of 1.5 GPa. The analysis of the relative displacements in Fig. 4b–d confirms that interface disconnections are 2 n -layer thick and no shear deformation is associated with the motion of interface disconnections. How to cite this article: Liu, B.-Y. et al. Twinning-like lattice reorientation without a crystallographic twinning plane. Nat. Commun. 5:3297 doi: 10.1038/ncomms4297 (2014).